Biexcitonic molecules survive excitons at the Mott transition When the carrier density is increased in a semiconductor, according to the predictions of Sir Nevil Mott, a transition should occur from an insulating state consisting of a gas of excitons to a conductive electron–hole plasma. This crossover, usually referred to as the Mott transition, is driven by the mutual effects of phase-space filling and Coulomb screening because of the presence of other charges nearby. It drastically affects the optical and electrical characteristics of semiconductors and may, for example, drive the transition from a polariton laser to a vertical cavity surface-emitting laser. Usually, the possible existence of excitonic molecules (or biexcitons) is neglected in the understanding of the Mott transition because the biexciton is supposed to be less robust against screening effects. Here, against common beliefs, we observe that the biexciton in a GaN quantum well is more stable towards the Mott transition than the exciton. The metal–insulator transition in electron–hole (e–h) systems, the so-called Mott transition (MT), has attracted a lot of interest over the years, both theoretically and experimentally [1] , [2] , [3] . The importance of the MT does not only arise from its close link with the onset of gain opening up the operation regime of conventional laser diodes but also stems from the fact that it marks the crossover from bosonic to fermionic quasi-particles in a semiconductor medium. Thus, it additionally sets the injection limit for the operation of polariton lasers [4] , [5] . Well-established theories exist for the dilute excitonic gas regime [6] as well as for the dense e–h plasma regime [7] . However, a theory that encompasses these two density regimes does not exist yet [8] . More interestingly, even if biexcitons (XX) are frequently seen to dominate the emission of semiconductor structures when the density is raised, and this is particularly true for GaN-based heterostructures [9] , no clear experimental report is available on the role of biexcitons in the MT in a two-dimensional (2D) nanostructure. A comprehensive study treating the MT in the presence of biexcitons can only be found for T-shaped GaAs-based quantum wires [10] . The generally accepted picture of the semiconductor MT follows the idea of a complex interplay between phase space-filling effects, the progressive broadening of the resonance via collisions, and the screening of Coulomb interactions between the exciton constituents, when the carrier density increases. Eventually, for a certain critical carrier density, the exciton energy coincides with the renormalized bandgap and the exciton resonance disappears within the broad response of the plasma. Although it is still debated whether the MT should be a first- or a second-order transition, experimental reports clearly favour the second option based on the absence of any observation of a sharp threshold [11] , [12] . A rough approximation for the Mott density corresponds to the inverse of the exciton volume [13] . In this approximation, the critical density for the injection-induced dissociation of biexcitons, is expected to be smaller than its excitonic counterpart owing to the larger biexciton Bohr radius [14] . Here we report on the crossover between a mixed exciton–biexciton gas and a conductive e–h plasma by probing a single GaN/AlGaN quantum well (QW) with picosecond time-resolved (TR) photoluminescence (PL). Our experiments directly address the dynamics and stability of biexcitons in the high carrier-density regime. Characteristics of the sample The studied sample consists of a polar 3-nm-thick single GaN QW sandwiched in between Al 0.05 Ga 0.95 N barriers. It was grown by metal organic vapour phase epitaxy on c -plane sapphire. More details on the growth can be found elsewhere [15] . As evidenced by PL excitation (PLE) measurements ( cf. Fig. 1a ), the optical density of the QW is governed by two narrow transitions (~5 meV linewidth), corresponding to the X A and X B excitons. The high structural quality is additionally confirmed by the small localization energy of ~1 meV, as deduced from a comparison between PLE and PL spectra in Fig. 1a . It allows us to observe and probe the transition of biexcitons that can be found on the low-energy side of the X A emission in Fig. 1a and that has been identified in a previous study on this sample [9] . Both transitions, X A and XX, can also be observed in the power-dependent continuous wave (CW) PL measurements ( Fig. 1b ) centred at 3.533 and 3.525 eV, respectively. The biexcitonic origin of the low-energy mode is consistent with the super-linear rise in the biexciton intensity in CW PL (see Fig. 1c ) and the thermalization dynamics in TR PL discussed below. Finally, we assign the emission lines around 3.560 and 3.48 eV to the luminescence of the 5% Al x Ga 1− x N barriers and the GaN buffer layer, respectively. Owing to the presence of intrinsic polarization fields in c -plane-oriented III-nitride heterostructures that lead to the quantum-confined Stark effect, the e–h wavefunction overlap may be markedly reduced in such QWs [16] . This effect is most prominent for low carrier densities, while increasing the latter will progressively screen the polarization field. Following the method described in ref. 5 , we employed self-consistent Schrödinger–Poisson (SP) simulations to model the density-dependent characteristics of the present QW structure with a built-in electric field of 180 kV cm −1 . We deduced an exciton-binding energy of ~30 meV from these SP simulations at zero carrier density in the QW. The biexciton-binding energy is estimated from the CW PL spectra under moderate injection to be ~8 meV. Hence, the ratio of the biexciton- to exciton-binding energy is ~0.26, that is, a value close to the 0.228 expected for weakly disordered structures [17] , [18] . 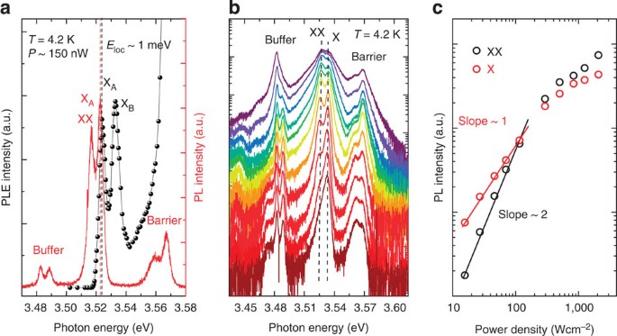Figure 1: PLE and power-dependent PL spectra of the sample. (a) PLE (black dots, solid line is a guide to the eye) and PL (red solid line) spectrum of the sample at moderate excitation. The localization energy ~1 meV is deduced by comparing the exciton energy in the PLE and the PL spectra. (b) Power-dependent PL spectra of the sample under CW laser excitation. The excitation power density changes from 3 up to 3,000 W cm−2from the lowest to the highest spectrum, respectively. (c) PL intensity of the exciton (red) and biexciton (black) peaks as a function of excitation power density. The linear and quadratic dependencies of the exciton and biexciton PL intensities at low injection confirm the assignment of these two peaks to excitons and biexcitons, respectively. Figure 1: PLE and power-dependent PL spectra of the sample. ( a ) PLE (black dots, solid line is a guide to the eye) and PL (red solid line) spectrum of the sample at moderate excitation. The localization energy ~1 meV is deduced by comparing the exciton energy in the PLE and the PL spectra. ( b ) Power-dependent PL spectra of the sample under CW laser excitation. The excitation power density changes from 3 up to 3,000 W cm −2 from the lowest to the highest spectrum, respectively. ( c ) PL intensity of the exciton (red) and biexciton (black) peaks as a function of excitation power density. The linear and quadratic dependencies of the exciton and biexciton PL intensities at low injection confirm the assignment of these two peaks to excitons and biexcitons, respectively. 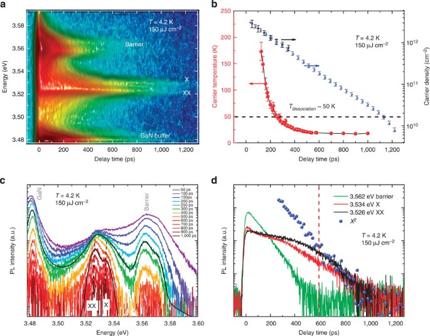Figure 2: TR PL measurements. (a) Streak image of the TR PL measurements taken at 4.2 K. The GaN buffer layer, exciton, biexciton and barrier emission energy are labelled. Note that the colour code was not provided because of the lightening effect that has been applied to enhance the visibility of the XX transition at longer delays. Panelcdisplays the quantitative data extracted from this streak image. (b) Extrapolated QW carrier density (blue) and carrier density values extracted from the e–h plasma modelling procedure at early time delays (black) as a function of the time delay after excitation. The error bars have been extracted according to the uncertainty in the fitting parameters such as the effective masses of electrons and holes. The correspondingly deduced effective carrier temperatures are shown in addition (red), with error bars showing the uncertainty induced by the inhomogeneous broadening. The black dashed line marks the temperature limit according to Saha’s law, where biexcitons are ionized according to their binding energy (8 meV). (c) TR PL spectra at different time delays from 50 to 1,000 ps in semilogarithmic scale atT=4.2 K. The estimated carrier density (in cm−2) in the QW corresponding to each spectrum from the upper to the lower one, respectively, is equal to: 2.83 × 1012, 2.20 × 1012, 1.73 × 1012, 1.37 × 1012, 1.07 × 1012, 8.40 × 1011, 5.02 × 1011, 3.00 × 1011, 1.85 × 1011, 1.16 × 1011, 7.51 × 1010, 4.96 × 1010and 3.22 × 1010. For the PL spectra taken at 250 and 600 ps time delay, fittings with the e–h plasma lineshape model and two Voigt functions are shown for comparison, respectively (black). (d) Decays of the PL intensity corresponding to the energy of the biexciton (3.526 eV), the exciton (3.534 eV) and the barrier (3.562 eV) in semilogarithmic scale. The square of the PL intensity at the exciton energy is also reported to show the thermodynamic equilibrium between excitons and biexcitons at long delays after the excitation. The red dashed line shows the delay time before thermodynamic equilibrium between excitons and biexcitons occurs. The small discrepancy in the energies of the QW between PLE and CW PL spectra, and also TR PL spectra, is because of small variations in the QW thickness along the sample. It was because of the fact that the growth of the well region was performed to produce a small wedge (cf.Supplementary Note 2). Full size image e–h plasma emission observation Figure 2a shows a representative streak image recorded in TR PL at 4.2 K. The PL spectrum measured 50 ps after the excitation pulse ( Fig. 2c ) features a characteristic plateau-like QW emission that extends from the biexciton emission energy continuously up to the barrier energy. The saturation of the emission amplitude at early delays is the direct signature of k -space filling of the constant 2D density-of-states and indicates the presence of a degenerate e–h plasma in the QW [19] . For the high-injection PL spectra at early time delays, that is within the first 300 ps, an e–h plasma lineshape fitting following the model discussed in refs 11 , 20 was employed ( cf. Supplementary Note 1 ). In order to extract absolute values for the QW carrier density n , A and B valence bands were considered to be energetically separated by 11 meV at k =0 according to PLE measurements, while effective electron and hole masses equal to , and , where m 0 denotes the free electron mass, were adopted as deduced from k.p simulations. Exemplarily, the result of this fitting procedure, based on a purely fermionic picture, is shown for the PL spectrum, taken 250 ps after excitation in Fig. 2c . In order to reproduce the full PL spectrum, the PL bands corresponding to the GaN buffer layer and the barrier have been modelled with additional Voigt functions. The very good agreement between modelling and experiment for time delays up to 300 ps ( cf. Supplementary Fig. 1 ) emphasizes the predominantly fermionic nature of recombining carriers in the high-density regime. Figure 2: TR PL measurements. ( a ) Streak image of the TR PL measurements taken at 4.2 K. The GaN buffer layer, exciton, biexciton and barrier emission energy are labelled. Note that the colour code was not provided because of the lightening effect that has been applied to enhance the visibility of the XX transition at longer delays. Panel c displays the quantitative data extracted from this streak image. ( b ) Extrapolated QW carrier density (blue) and carrier density values extracted from the e–h plasma modelling procedure at early time delays (black) as a function of the time delay after excitation. The error bars have been extracted according to the uncertainty in the fitting parameters such as the effective masses of electrons and holes. The correspondingly deduced effective carrier temperatures are shown in addition (red), with error bars showing the uncertainty induced by the inhomogeneous broadening. The black dashed line marks the temperature limit according to Saha’s law, where biexcitons are ionized according to their binding energy (8 meV). ( c ) TR PL spectra at different time delays from 50 to 1,000 ps in semilogarithmic scale at T =4.2 K. The estimated carrier density (in cm −2 ) in the QW corresponding to each spectrum from the upper to the lower one, respectively, is equal to: 2.83 × 10 12 , 2.20 × 10 12 , 1.73 × 10 12 , 1.37 × 10 12 , 1.07 × 10 12 , 8.40 × 10 11 , 5.02 × 10 11 , 3.00 × 10 11 , 1.85 × 10 11 , 1.16 × 10 11 , 7.51 × 10 10 , 4.96 × 10 10 and 3.22 × 10 10 . For the PL spectra taken at 250 and 600 ps time delay, fittings with the e–h plasma lineshape model and two Voigt functions are shown for comparison, respectively (black). ( d ) Decays of the PL intensity corresponding to the energy of the biexciton (3.526 eV), the exciton (3.534 eV) and the barrier (3.562 eV) in semilogarithmic scale. The square of the PL intensity at the exciton energy is also reported to show the thermodynamic equilibrium between excitons and biexcitons at long delays after the excitation. The red dashed line shows the delay time before thermodynamic equilibrium between excitons and biexcitons occurs. The small discrepancy in the energies of the QW between PLE and CW PL spectra, and also TR PL spectra, is because of small variations in the QW thickness along the sample. It was because of the fact that the growth of the well region was performed to produce a small wedge ( cf. Supplementary Note 2 ). Full size image For the purpose of estimating the carrier density at longer delays ( cf. Fig. 2b ), the carrier concentration deduced from the modelling procedure was scaled for each time delay based on the overall captured QW emission intensity in the streak image according to: I PL ∝ d n /d t . More precisely, for each point in time the carrier density results from the initial carrier concentration multiplied by the integrated intensity of the streak image, which was summed spectrally over the QW emission and temporally between the considered time step and infinity ( cf. ref. 11 ). Owing to the high quality of the structure, we assumed a negligible contribution of nonradiative recombination at low temperature. This step allows us to transpose the TR measurements into carrier density-dependent spectra. Emergence of e–h plasma emission from the biexcitons The maximum carrier density in the QW, determined 50 ps after the excitation, amounts to ~3 × 10 12 cm −2 , the latter being basically limited by the finite barrier height. Within the first 300 ps, the radiative decay of the carrier concentration induces a gradual shrinkage of the QW emission plateau on its high-energy side, while the PL amplitude on the low-energy side stays almost constant. This saturation of the PL intensity at early time delays because of phase space filling can also be followed when comparing the temporal evolution of the emission intensity at the exciton and biexciton energies in Fig. 2d . Interestingly, after the first 300 ps a clear peak at the biexciton energy appears, while the high-energy tail of the QW emission remains purely exponential, still indicating the fermionic nature of the carriers at the Fermi energy [11] . Only at even longer delays and thus for a further decrease in carrier density, another peak appears at the exciton energy. In this regime, the PL spectrum is well reproduced by two Voigt functions for the exciton and biexciton transitions, as shown at 600-ps time delay in Fig. 2c , evidencing the dominant role of excitons in this low-injection regime. This interpretation is fully supported by the PL transients displayed in Fig. 2d : for time delays longer than 600 ps, the biexciton PL intensity follows the squared slope of the exciton intensity, which indicates thermal equilibrium between exciton and biexciton populations [21] . To rephrase our findings, up to carrier densities of 5 × 10 11 cm −2 , the emission properties of the present GaN QWs are dominated by excitonic recombination. A further increase in carrier density first leads to the vanishing of the exciton line in the high-energy shoulder of the biexciton emission band, and eventually to the observation of a broad e–h plasma emission at densities in excess of 1 × 10 12 cm −2 . The latter is evidenced by the saturation of the PL intensity amplitude at high densities and a characteristic asymmetric emission lineshape, which can be accurately modelled using Fermi’s golden rule. Similarly to experiments conducted in GaAs-based QWs, the MT appears to be smooth [17] . However, contrary to the GaAs system, here the e–h plasma builds up from the biexciton state rather than from the exciton resonance. Moreover, when the carrier density in the QW increases, the excitonic resonance seems to disappear at lower injection than does the biexcitonic one. This observation is contrasting with the intuitive expectation exposed above: high-density effects are supposed to first screen the biexciton resonance, owing to its larger Bohr radius and smaller binding energy [14] , [17] . 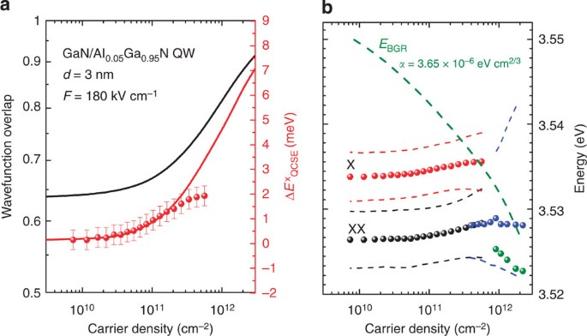Figure 3: Self-consistent SP simulation results, exciton and biexciton emission energy and broadening, and BGR as a function of injected carrier density in the QW. (a) Results of SP simulations for the e–h wavefunction overlap (black curve) and shift in exciton energy because of screening of the built-in electric field in the QW (red solid curve) compared with the experimental values of the exciton emission energy shift (red circles). The error bars are the standard deviations of the fitting of experimental data with two Voigt functions for excitons and biexcitons. (b) Energy of the exciton and biexciton transitions (red and black circles, respectively) in addition to their full-width at half-maximum (FWHM) energies (shown by dashed lines) as a function of the QW carrier density. The energy difference between exciton and biexciton energies, that is, the biexciton-binding energy, remains constant over the entire power density range. The green circles represent the values of the bandgap extracted from e–h plasma emission modelling. Beyond the MT, the QW emission peak and FWHM energies are shown with blue dots and dashed lines, respectively. It is obvious that they emerge from the biexciton emission band. The green dashed line shows the expected evolution of the band edge because of BGR withα=3.65 × 10−6eV cm2/3in agreement with refs20,22. Determination of the critical carrier density Figure 3b shows the QW emission characteristics, that is, peak energies and emission linewidths, as a function of the determined carrier density. An increase in n from 7 × 10 9 to 5 × 10 11 cm −2 leads to an exciton emission energy blueshift by ~2 meV. This effect can quite accurately be reproduced by SP simulations accounting for the screening of the built-in electric field (see Fig. 3a ): it leads to a blueshift of the QW transition energy Δ E QW ( n ) and an increase in the e–h wavefunction overlap. The latter raises from a zero-density value of 0.64 to ~0.81 at a carrier density of 1 × 10 12 cm −2 , which simultaneously causes an increase in the exciton-binding energy. Eventually, the density dependence of the exciton energy can be written as: Figure 3: Self-consistent SP simulation results, exciton and biexciton emission energy and broadening, and BGR as a function of injected carrier density in the QW. ( a ) Results of SP simulations for the e–h wavefunction overlap (black curve) and shift in exciton energy because of screening of the built-in electric field in the QW (red solid curve) compared with the experimental values of the exciton emission energy shift (red circles). The error bars are the standard deviations of the fitting of experimental data with two Voigt functions for excitons and biexcitons. ( b ) Energy of the exciton and biexciton transitions (red and black circles, respectively) in addition to their full-width at half-maximum (FWHM) energies (shown by dashed lines) as a function of the QW carrier density. The energy difference between exciton and biexciton energies, that is, the biexciton-binding energy, remains constant over the entire power density range. The green circles represent the values of the bandgap extracted from e–h plasma emission modelling. Beyond the MT, the QW emission peak and FWHM energies are shown with blue dots and dashed lines, respectively. It is obvious that they emerge from the biexciton emission band. The green dashed line shows the expected evolution of the band edge because of BGR with α =3.65 × 10 −6 eV cm 2/3 in agreement with refs 20 , 22 . Full size image Note, however, that exciton screening and phase space filling are not considered in these SP calculations. As a consequence, we observe a deviation of the exciton blueshift from the SP prediction when exceeding concentrations of 3 × 10 11 cm −2 in Fig. 3a . Indeed, it is expected that the quantum-confined Stark effect screening effects on either the QW transition-energy blueshift or the increasing exciton-binding energy are going to be overcompensated by saturation effects when approaching the MT. In addition, a slight increase in the PL linewidth for both the exciton and the biexciton is observed at similar densities in Fig. 3b , which can be ascribed to collisional-induced broadening [19] . Figure 3b also depicts the determined bandgap energy that characteristically shifts to lower energy with increasing n because of bandgap renormalization (BGR). The carrier density dependence of the bandgap energy E BGR is commonly described by [20] , [22] : where α denotes a material and dimensionality dependent constant, which was chosen to be equal to 3.65 × 10 −6 eV cm 2/3 in agreement with refs 20 , 22 . The predicted evolution matches the experimental points and leads to an estimate for the critical density of ~6 × 10 11 cm −2 , given by the intersection between E BGR and E X ( n ). This criterion corresponds to the vanishing of the exciton-binding energy and is in good agreement with the spectral analysis given before. Density independence of the biexciton-binding energy According to the aforementioned analysis of BGR, the exciton-binding energy tends to be zero when the carrier density approaches the critical limit for the MT. Assuming that Haynes rule [18] is still valid at these carrier densities, a pronounced decrease in the biexciton-binding energy would also be expected. However, we observe almost no change in the energy difference between the exciton and the biexciton transitions ( Fig. 3b ), that is, the biexciton-binding energy, which implies a remarkable stability of biexcitons at high carrier densities. Moreover, when following the peak and half-maximum energies of the QW emission above the MT shown in Fig. 3b (blue dots and blue dashed lines, respectively), it is obvious that in presence of an increasing carrier density the e–h plasma emission directly emerges from the biexciton emission band. At the first sight, the robustness of biexcitonic molecules might seem surprising if one considers their smaller binding energy compared with that of excitons. However, this could originate from the complex interplay between correlation and exchange processes occurring in those molecules built from four particles when interacting with nearby carriers. Since the existence of biexcitons was neglected in most of theoretical lines of work accounting for a varying carrier density, likely because of their reduced stability in smaller bandgap QW heterostructures such as GaAs, our results call for more theoretical investigations considering the important role that can be played by those quasi-particles at the MT. However, our results can also be understood by applying Saha’s law to excitons and biexcitons [21] . In such a case, the biexciton is expected to be the predominant species at high injection. The absence of any biexcitonic transition at high carrier densities in GaAs heterostructures could be because of the fact that, when increasing the carrier density, the temperature of the exciton gas is also raised. Considering the low binding energy of biexcitons in GaAs (1.5 meV [17] ), biexcitons are expected to get ionized once the excitonic gas temperature exceeds 20 K. However, in the GaN-based structures studied here, biexcitons can survive at temperatures up to 50 K, thanks to their large binding energy of 8 meV. As shown in Fig. 2b , owing to efficient phonon-cooling, the effective carrier temperature in our measurements remains below 50 K up to carrier densities ~10 12 cm −2 , which allows the formation of biexcitons. In conclusion, our experimental results as a function of carrier density show a crossover from excitons to biexcitons and finally to an e–h plasma in a 2D system. The emergence of the e–h plasma emission spectrum directly from the biexciton energy reveals the important role played by biexcitons in the MT. Thereby, the stability of biexciton molecules against Coulomb-screening and collisions is evidenced by the invariance of the biexciton-binding energy up to the critical density. Although the possibility of a transition from an e–h plasma directly to a biexciton gas for a one dimensional (1D) system was predicted in ref. 2 within a two-band Hubbard model, biexcitons were not considered in most of the theoretical lines of work up to now. Hence, our work opens up new perspectives to revisit the theoretical framework of stability of biexciton molecules in the high-density regime. Continuous-wave and TR PL measurements To study the sample at high carrier injection, both CW PL and TR PL experiments have been performed. Power-dependent CW PL spectra have been recorded by exciting the sample with a frequency-doubled Ar + -laser ( λ =244 nm). For TR PL experiments, the sample was excited with the third harmonic ( λ =280 nm) of a picosecond mode-locked Ti:sapphire laser. The excitation beam is focused on the sample by means of a 2.5-mm-focal length UV objective (NA=0.55) that allows for an excitation spot diameter below 5 μm. A key issue for the present measurements, where the luminescence signal critically depends on the excitation power density, is to carefully position a spatial filter in the collection path. For this purpose, the centre of the PL spot on the sample was magnified 100 times and sent through a 50-μm pinhole placed in the collection line, which allowed us to probe a region with a uniform excitation density. This spatial filtering step in the collection line is of crucial importance, since it avoids the contribution of a wide range of carrier densities in the PL signal and enhances the clarity of the measurements. The collected PL was spectrally and temporally analysed using a 32-cm-focal length monochromator equipped with a CCD (charge-coupled device) and a streak camera. A 1,200-groove per mm grating was used to disperse the PL spectra, which allows us to reach a spectral resolution better than 1 meV. For the TR analysis, the streak camera was used with a temporal resolution of ~5 ps in synchronous scan mode. Fitting of the exciton and biexciton PL spectra Figure 3a,b shows the exciton and biexciton emission energy as well as their full-width at half-maximum as a function of carrier density. The data points are the results of fitting of the spectra with two Voigt profiles for carrier densities below 6 × 10 11 cm −2 . The Gaussian broadening was estimated from the PL spectrum taken at very low carrier density and then kept constant while fitting the PL spectra at higher carrier densities. For carrier densities larger than 6 × 10 11 cm −2 , the QW emission shows an increase in the slope on its high-energy tail. It was therefore not possible to apply the same fitting procedure with two simple Voigt functions for the PL spectra beyond those densities. In order to handle the increasing noise at long time delays, the measurement shown in Fig. 2a was repeated under identical conditions with longer integration time, leading to an overexposition at early delays. How to cite this article: Shahmohammadi, M. et al. Biexcitonic molecules survive excitons at the Mott transition. Nat. Commun. 5:5251 doi: 10.1038/ncomms6251 (2014).